Tamoxifen augments the innate immune function of neutrophils through modulation of intracellular ceramide Tamoxifen is a selective oestrogen receptor modulator widely used for the treatment of breast cancer. In addition to its activity as an oestrogen receptor agonist/antagonist, tamoxifen also modulates sphingolipid biosynthesis, which has been shown to play an important role in the regulation of neutrophil activity. Here, we find that tamoxifen stimulation enhances several pro-inflammatory pathways in human neutrophils, including chemotaxis, phagocytosis and neutrophil extracellular trap (NET) formation. The enhancement of NET production occurs via a ceramide/PKCζ-mediated pathway, and treatment with synthetic ceramide is sufficient to promote NET formation. Pretreatment of human neutrophils with tamoxifen boosts neutrophil bactericidal capacity against a variety of pathogens in vitro and enhances clearance of the leading human pathogen methicillin-resistant Staphylococcus aureus in vivo . Our results suggest that tamoxifen, and the lipid signalling pathways it modulates, merit further exploration as targets for boosting host innate immune function. Tamoxifen, a selective oestrogen receptor modulator taken by hundreds of thousands of patients for the treatment of breast cancer [1] , is included on the World Health Organization’s list of essential medicines due to its cost effectiveness and safety profile [2] . In addition to its activity as an oestrogen receptor agonist/antagonist [3] , tamoxifen has many other effects that include modulation of sphingolipid biosynthesis [4] . Such ‘off-target’ effects have been shown to contribute to the therapeutic action of tamoxifen [5] ; however, its impact on some normally functioning cell types, in particular circulating neutrophils, remains poorly understood. Earlier investigations of the impact of tamoxifen on neutrophil function have largely been limited to its inhibition of transendothelial migration, suggesting a primary immunosuppressant activity [6] , [7] . Because sphingolipids are known to be important modulators of immune cell function [8] , we investigated the effects of tamoxifen on human neutrophils, the primary phagocytic leukocyte of the immune system. Using in vitro and in vivo approaches, we find that tamoxifen, in addition to enhancing neutrophil chemotaxis and phagocytosis, strongly promotes the formation of DNA-based neutrophil extracellular traps (NETs). NETs, which are coated with antimicrobial peptides, histones and/or granule proteases, are capable of entrapping and killing bacteria and other pathogens [9] , [10] . Tamoxifen enhances killing of pathogens in vitro and enhances clearance of methicillin-resistant Staphylococcus aureus (MRSA) in vivo . We find that such alterations in neutrophil activity are dependent on intracellular ceramide. Direct assessment of N -Formyl-Met-Leu-Phe (fMLP)-induced neutrophil chemotaxis indicated that tamoxifen, while not stimulating chemotaxis by itself ( Supplementary Fig. 1 ), significantly enhanced directional cell migration in response to fMLP stimulation ( Fig. 1a ). These differences in findings may be due to variations in protocol (for example, previous studies pre-incubated cells with tamoxifen and removed it before assessment of chemotaxis rather than assessing migration in its presence) or the added complexity of in vitro transendothelial migration models. In addition to these findings, fluorescence-based quantification of extracellular DNA release revealed that tamoxifen ( Fig. 1b ), its active metabolite 4-hydroxytamoxifen ( Fig. 1b ) and its primary metabolite N -desmethyltamoxifen ( Supplementary Fig. 2 ), strongly stimulated NET production in freshly isolated human neutrophils. These results were confirmed by immunostaining of stimulated neutrophils using a primary antibody against myeloperoxidase, a NET marker ( Fig. 1c ) [11] . Because tamoxifen is generally described to have antagonist activity at the oestrogen nuclear receptors ERα and ERβ and agonist activity at the G-protein-coupled oestrogen receptor GPR30, we attempted to replicate these results using selective agonists/antagonists. In these studies, NET production was not observed in response to treatment with Methyl-piperidino-pyrazole (MPP) or pyrazolo [1,5-a] pyrimidine (PHTPP) (selective ERα and ERβ antagonists, respectively [12] , [13] ), G-1 (a GPR30 agonist [14] ) or fulvestrant (a selective oestrogen receptor modulator that mimics the mixed agonist/antagonist characteristics of tamoxifen [15] , [16] ) ( Supplementary Fig. 3 ), indicating that tamoxifen-induced NET production is mediated by an oestrogen receptor-independent mechanism. 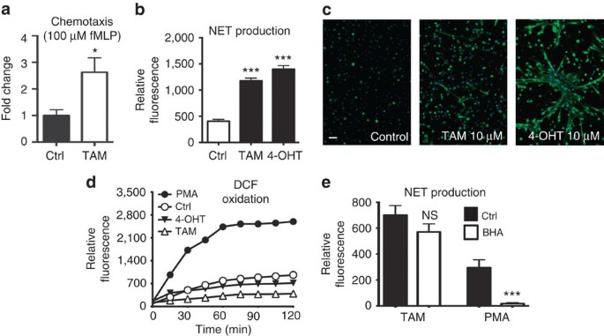Figure 1: Tamoxifen promotes extracellular trap formation in human neutrophilsin vitro. (a) The effect of 10 μM tamoxifen (TAM; upper well) on chemotaxis in the presence or absence of 100 nM fMLP (lower well) was determined using a transwell system (n=12). (b) Extracellular DNA was quantified to determine the effect of both TAM and 4-hydroxytamoxifen (4-OHT) on NET release (n=9). (c) NET production was confirmed by fixing and immunostaining TAM-/4-OHT-stimulated cells with DAPI and a primary antibody for myeloperoxidase (blue: DAPI; green: NETs/myeloperoxidase); images representative of three independent experiments shown (scale bar=50 μm). (d) DCF-based ROS assays were performed to evaluate the effect of TAM and 4-HT on ROS production (n=9). (e) Neutrophils were pre-incubated with the ROS scavenger BHA before addition of either PMA to TAM to determine whether ROS production is required for tamoxifen-induced NET production (n=9). Where applicable, results were analysed by one-way analysis of variance and post hoc Newman Keuls test. *P<0.05, ***P<0.001 versus control values. BHA, butylated hydroxyanisole; DAPI, 4′,6-diamidino-2-phenylindole; NS, not significant; ROS, reactive oxygen species. Figure 1: Tamoxifen promotes extracellular trap formation in human neutrophils in vitro . ( a ) The effect of 10 μM tamoxifen (TAM; upper well) on chemotaxis in the presence or absence of 100 nM fMLP (lower well) was determined using a transwell system ( n =12). ( b ) Extracellular DNA was quantified to determine the effect of both TAM and 4-hydroxytamoxifen (4-OHT) on NET release ( n =9). ( c ) NET production was confirmed by fixing and immunostaining TAM-/4-OHT-stimulated cells with DAPI and a primary antibody for myeloperoxidase (blue: DAPI; green: NETs/myeloperoxidase); images representative of three independent experiments shown (scale bar=50 μm). ( d ) DCF-based ROS assays were performed to evaluate the effect of TAM and 4-HT on ROS production ( n =9). ( e ) Neutrophils were pre-incubated with the ROS scavenger BHA before addition of either PMA to TAM to determine whether ROS production is required for tamoxifen-induced NET production ( n =9). Where applicable, results were analysed by one-way analysis of variance and post hoc Newman Keuls test. * P <0.05, *** P <0.001 versus control values. BHA, butylated hydroxyanisole; DAPI, 4′,6-diamidino-2-phenylindole; NS, not significant; ROS, reactive oxygen species. Full size image To elucidate the pathway underlying the neutrophil-activating effects of tamoxifen, we next assessed signalling molecules/effectors typically associated with NET release. Although NET production has been reported to be dependent on reactive oxygen species (ROS) generation [17] , we found that both tamoxifen and 4-hydroxytamoxifen lowered ROS production in human neutrophils ( Fig. 1d ), mirroring our previous findings with statins [18] . This finding was supported by experiments using the ROS scavenger butylated hydroxyanisole, which potently inhibited phorbol myristate acetate (PMA)-induced NET production, but did not significantly reduce tamoxifen-induced NET production ( Fig. 1e ). In contrast, pre-incubation with the general PKC antagonist chelerythrine chloride inhibited tamoxifen-induced NET production ( Fig. 2a ). To determine the specific PKC isoform responsible for tamoxifen-induced NET release, we stimulated neutrophils with tamoxifen in the presence of two broad-spectrum PKC inhibitors with different selectivity profiles, Gö 6973 and Gö 6983, the latter of which is a more potent inhibitor of PKCζ and PKCμ (ref. 19 ). Inhibition curves revealed that Gö 6983 exhibited greater inhibition of tamoxifen-induced NET production, pointing to either PKCζ or PKCμ as the primary PKC isoform responsible for this induction ( Fig. 2b ). Further experiments using a highly selective inhibitor of PKCζ, PKCζ pseudosubstrate (PKCζ-PS) [20] , resulted in near-complete inhibition of tamoxifen-induced NET production, strongly implicating PKCζ as a key mediator of this process ( Fig. 2c ). Inhibition of PI3K had no effect on tamoxifen-induced NET production ( Supplementary Fig. 4 ), although tamoxifen promoted translocation of neutrophil PKCζ ( Fig. 2d ). The importance of PKCζ in tamoxifen-induced NET production was confirmed in experiments using bone marrow-derived neutrophils collected from PKCζ knockout animals, which showed significantly reduced NET production following tamoxifen treatment compared with wild-type littermate controls ( Fig. 2e ). 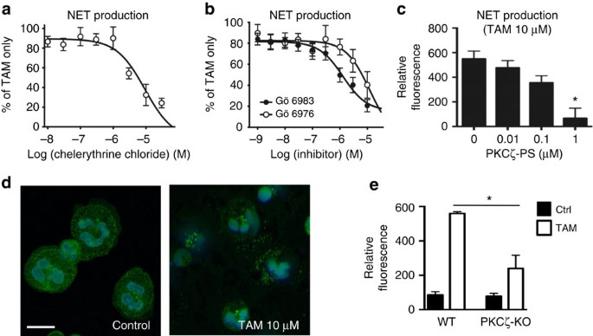Figure 2: Tamoxifen-induced extracellular trap production is PKCζ dependent. (a) To determine whether PKC is required for TAM-induced NET production, neutrophils were pre-incubated with (a) the general PKC antagonist chelerythrine chloride (n=8) or (b) the more selective inhibitors Gö 6976 and Gö 6983 (n=9) before treatment with 10 μM TAM. (c) Neutrophils were pre-incubated with PKCζ pseudosubstrate (PKCζ-PS) to specifically evaluate the role of PKCζ in TAM-induced NET production. (d) Immunostaining/confocal microscopy was used to visualize translocation of PKCζ in human neutrophils in response to TAM (10 μM) treatment (blue: 4′,6-diamidino-2-phenylindole; green: PKCζ); images representative of three independent experiments are shown (scale bar, 10 μm). (e) Bone marrow-derived neutrophils were collected from PKCζ knockout mice to determine TAM-induced NET production in comparison with wild-type (WT) littermate controls (n=4–5). Where applicable, results were analysed by one-way analysis of variance andpost hocNewman Keuls test. *P<0.05 versus control values. Figure 2: Tamoxifen-induced extracellular trap production is PKCζ dependent. ( a ) To determine whether PKC is required for TAM-induced NET production, neutrophils were pre-incubated with ( a ) the general PKC antagonist chelerythrine chloride ( n =8) or ( b ) the more selective inhibitors Gö 6976 and Gö 6983 ( n =9) before treatment with 10 μM TAM. ( c ) Neutrophils were pre-incubated with PKCζ pseudosubstrate (PKCζ-PS) to specifically evaluate the role of PKCζ in TAM-induced NET production. ( d ) Immunostaining/confocal microscopy was used to visualize translocation of PKCζ in human neutrophils in response to TAM (10 μM) treatment (blue: 4′,6-diamidino-2-phenylindole; green: PKCζ); images representative of three independent experiments are shown (scale bar, 10 μm). ( e ) Bone marrow-derived neutrophils were collected from PKCζ knockout mice to determine TAM-induced NET production in comparison with wild-type (WT) littermate controls ( n =4–5). Where applicable, results were analysed by one-way analysis of variance and post hoc Newman Keuls test. * P <0.05 versus control values. Full size image Through its ability to inhibit glucosylceramide synthase, a key enzyme in the sphingolipid synthesis pathway that converts ceramide to glucosylceramide, tamoxifen has been shown in some cell types to promote intracellular accumulation of ceramide, a potent PKCζ activator [21] . Thus, we next determined whether ceramide accumulation could drive tamoxifen-induced NET production. Indeed, similar to tamoxifen, ceramide promoted NET release in a concentration-dependent manner ( Fig. 3a,b ) while inhibiting ROS generation ( Fig. 3c ). Ceramide-induced NET production was also PKC/PKCζ dependent ( Fig. 3d ). Mass spectrometry revealed a statistically significant increase in C16 and C24 ceramide species in neutrophils upon tamoxifen treatment. Structural verification of ceramide species was obtained with high mass accuracy of the parent ion and additionally by monitoring the hallmark 264-Dalton ion fragment released during the fragmentation of ceramides via tandem mass spectrometry ( Fig. 3e ; Supplementary Fig. 5 ). Elevated intracellular ceramides were also visually confirmed via immunocytochemistry using an anti-ceramide antibody ( Fig. 3f ). Further evidence of the role of ceramide in NET production was obtained by treating cells with D,L-threo-1-phenyl-2-decanoylamino-3-morpholino-1-propanol (DL-PDMP), a selective inhibitor of glucosylceramide synthase that mimics the intracellular ceramide-increasing effect of tamoxifen [22] , which also promoted NET production ( Fig. 3g ). Sphingosine-1-phosphate, which is generated from ceramide via the cascade initiated by glucosylceramide synthase [23] , did not significantly promote NET production ( Supplementary Fig. 6 ). To further confirm that tamoxifen-induced NET production is ceramide dependent, we pre-incubated neutrophils with myriocin, an inhibitor of serine palmitoyltransferase [24] . Inhibition of this enzyme, which initiates the pathway that generates ceramide from palmitoyl-CoA, prevents tamoxifen-mediated ceramide accumulation [25] . Although it does not directly inhibit PKCζ ( Supplementary Fig. 7 ), myriocin treatment resulted in complete inhibition of tamoxifen-induced NET production ( Fig. 3h ) and partially reversed inhibition of PMA-induced ROS production by tamoxifen ( Supplementary Fig. 8 ), illustrating the key role of ceramide accumulation in this pathway. 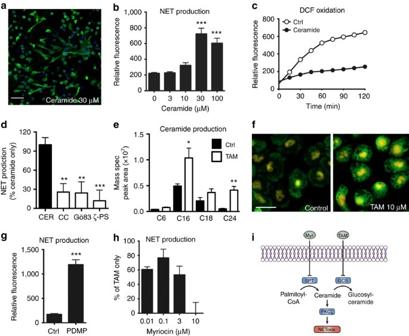Figure 3: Tamoxifen-induced NET production is mediated by intracellular ceramide. (a) Ceramide-induced NET production was visualized by immunostaining neutrophils for myeloperoxidase (blue: DAPI; green: NETs/myeloperoxidase); images representative of three independent experiments are shown (scale bar, 50 μm). (b) Quantification of extracellular DNA/NET production in response to ceramide treatment (n=9). (c) The effect of ceramide (30 μM) on ROS production was determined using DCF-based ROS assays (n=9). (d) Neutrophils were pre-incubated with PKC inhibitors (CC=chelerythrine chloride, Gö83=Gö 6983, ζ-PS=PKCζ pseudosubstrate; 10 μM each;n=9) to determine the involvement of PKC in ceramide-induced NET production. (e) Mass spectrometry analysis of lipid extracts was performed to quantify intracellular accumulation of several ceramide species in response to TAM treatment (10 μM). (f) Intracellular ceramide levels in control and TAM-treated (10 μM) neutrophils were visualized via immunostaining of fixed neutrophils using a ceramide primary antibody (green: ceramide); images representative of three independent experiments are shown, with identical exposure and gain settlings used for control and TAM-treated samples (scale bar, 20 μm). (g) The effect of DL-PDMP, which similar to tamoxifen inhibits glucosylceramide synthase, on NET production was assessed via quantification of extracellular DNA (n=9). (h) Myriocin, which blocks ceramide synthesis by inhibiting serine palmitoyltransferase, concentration dependently inhibits tamoxifen-induced NET production. (i) Summary of the mechanism of tamoxifen-induced NET production. By inhibiting glucosylceramide synthase, tamoxifen treatment leads to an accumulation of neutrophil intracellular ceramide levels, which promotes NET formation via activation of PKCζ. Where applicable, results were analysed by one-way analysis of variance andpost hocNewman Keuls test. *P<0.05, **P<0.01, ***P<0.001 versus control values. ROS, reactive oxygen species. Figure 3: Tamoxifen-induced NET production is mediated by intracellular ceramide. ( a ) Ceramide-induced NET production was visualized by immunostaining neutrophils for myeloperoxidase (blue: DAPI; green: NETs/myeloperoxidase); images representative of three independent experiments are shown (scale bar, 50 μm). ( b ) Quantification of extracellular DNA/NET production in response to ceramide treatment ( n =9). ( c ) The effect of ceramide (30 μM) on ROS production was determined using DCF-based ROS assays ( n =9). ( d ) Neutrophils were pre-incubated with PKC inhibitors (CC=chelerythrine chloride, Gö83=Gö 6983, ζ-PS=PKCζ pseudosubstrate; 10 μM each; n =9) to determine the involvement of PKC in ceramide-induced NET production. ( e ) Mass spectrometry analysis of lipid extracts was performed to quantify intracellular accumulation of several ceramide species in response to TAM treatment (10 μM). ( f ) Intracellular ceramide levels in control and TAM-treated (10 μM) neutrophils were visualized via immunostaining of fixed neutrophils using a ceramide primary antibody (green: ceramide); images representative of three independent experiments are shown, with identical exposure and gain settlings used for control and TAM-treated samples (scale bar, 20 μm). ( g ) The effect of DL-PDMP, which similar to tamoxifen inhibits glucosylceramide synthase, on NET production was assessed via quantification of extracellular DNA ( n =9). ( h ) Myriocin, which blocks ceramide synthesis by inhibiting serine palmitoyltransferase, concentration dependently inhibits tamoxifen-induced NET production. ( i ) Summary of the mechanism of tamoxifen-induced NET production. By inhibiting glucosylceramide synthase, tamoxifen treatment leads to an accumulation of neutrophil intracellular ceramide levels, which promotes NET formation via activation of PKCζ. Where applicable, results were analysed by one-way analysis of variance and post hoc Newman Keuls test. * P <0.05, ** P <0.01, *** P <0.001 versus control values. ROS, reactive oxygen species. Full size image Having established that tamoxifen stimulates neutrophil migration and induces NET production, we examined whether neutrophil bactericidal capacity could be enhanced via tamoxifen treatment. At the concentrations used to stimulate neutrophils, tamoxifen and 4-hydroxytamoxifen had negligible effects on the growth of the USA300 strain of community-associated MRSA, Escherichia coli (K1 serotype) or Pseudomonas aeruginosa (PA01 strain) ( Fig. 4a ). However, both tamoxifen and 4-hydroxytamoxifen enhanced the killing activity of activated human neutrophils against unopsonized bacteria of all three species ( Fig. 4b ). Treatment of neutrophils with ceramide mimicked these effects ( Supplementary Fig. 9 ). Live/dead staining of USA300 MRSA exposed to either control or tamoxifen-treated neutrophils revealed dead bacteria within the NETs of stimulated neutrophils, in contrast to mostly live bacteria surrounding the untreated neutrophils producing fewer NETs ( Fig. 4c ). Addition of DNAse to neutrophils before the addition of bacteria significantly enhanced bacterial recovery ( Fig. 4d ), suggesting that the bactericidal effects of tamoxifen are largely NET driven. Addition of DNase to neutrophil/bacteria culture samples before serial dilution and plating indicated that reductions in colony-forming units (CFUs) were primarily due to killing, rather than clumping, of bacteria ( Supplementary Fig. 10 ). Several different approaches confirmed that the DNAse used in these experiments was active, being able to both degrade DNA and eliminate NETs ( Supplementary Fig. 11 ). Given that some reports have suggested that the principal activity of NETs is to clump rather than kill bacteria [26] , [27] , our results provide evidence that NETs are heterogeneous in both their mechanism of formation and activity. Both tamoxifen and 4-hydroxytamoxifen also stimulated the uptake of S. aureus -labelled bioparticles ( Supplementary Fig. 12 ), suggesting a further activity to upregulate phagocytic pathways. Additional experiments using USA300 MRSA opsonized by incubation in pooled human serum also revealed enhanced bactericidal activity of neutrophils following a 10-min pre-incubation with tamoxifen ( Fig. 4e ). 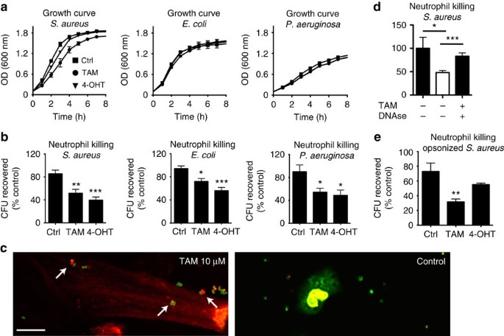Figure 4: Tamoxifen enhances neutrophil killing. (a) Bacterial growth curves for USA300 methicillin-resistantStaphylococcus aureus(MRSA), K1 strainE. colior PA01 strainP. aeruginosa(n=6) in the presence or absence of 10μM TAM or 4-hydroxytamoxifen (4-OHT). (b) Bactericidal assays evaluating the effect of a 4-h TAM or 4-OHT pre-treatment on neutrophil killing (represented by a reduction of CFUs) of USA300 MRSA,E. coliandP. aeruginosa(n=9–12). (c) Live/dead cell analysis of fixed cells; dead bacteria (red: propidium iodide, indicated by arrows) can be observed in tamoxifen-stimulated NETs (left panel). Live bacteria (green: SYTO 8) can be observed outside of the NETs and surrounding unstimulated cells (right panel). Images shown are representative of three independent experiments (scale bar, 10 μm). (d) Addition of DNAse before addition of bacteria to tamoxifen-treated neutrophils significantly reduces killing (n=9). (e) Neutrophils were incubated with TAM and bacteria concurrently to determine killing of USA300 MRSA opsonized using pooled human serum (n=8–9). Where applicable, results were analysed by one-way analysis of variance andpost hocNewman Keuls test. *P<0.05, **P<0.01, ***P<0.001 versus control values. Figure 4: Tamoxifen enhances neutrophil killing. ( a ) Bacterial growth curves for USA300 methicillin-resistant Staphylococcus aureus (MRSA), K1 strain E. coli or PA01 strain P. aeruginosa ( n =6) in the presence or absence of 10μM TAM or 4-hydroxytamoxifen (4-OHT). ( b ) Bactericidal assays evaluating the effect of a 4-h TAM or 4-OHT pre-treatment on neutrophil killing (represented by a reduction of CFUs) of USA300 MRSA, E. coli and P. aeruginosa ( n =9–12). ( c ) Live/dead cell analysis of fixed cells; dead bacteria (red: propidium iodide, indicated by arrows) can be observed in tamoxifen-stimulated NETs (left panel). Live bacteria (green: SYTO 8) can be observed outside of the NETs and surrounding unstimulated cells (right panel). Images shown are representative of three independent experiments (scale bar, 10 μm). ( d ) Addition of DNAse before addition of bacteria to tamoxifen-treated neutrophils significantly reduces killing ( n =9). ( e ) Neutrophils were incubated with TAM and bacteria concurrently to determine killing of USA300 MRSA opsonized using pooled human serum ( n =8–9). Where applicable, results were analysed by one-way analysis of variance and post hoc Newman Keuls test. * P <0.05, ** P <0.01, *** P <0.001 versus control values. Full size image We next tested tamoxifen in a murine model of systemic MRSA infection. At 1 h following intraperitoneal (i.p.) treatment with tamoxifen or vehicle control (corn oil), outbred CD-1 mice were infected i.p. with a lethal dose of USA300 MRSA. Mice were subsequently treated with tamoxifen or vehicle control at 1 and 8 h post infection. Tamoxifen provided significant protection against mortality ( Fig. 5a ); whereas all mice in the control group died on day 1, 40% of the tamoxifen-treated mice remained alive at day 3 and 33% surviving to the experimental end point (5 days). In subsequent experiments, mice were treated with tamoxifen or vehicle 2 h before and 6 h after i.p. infection with an enhanced green fluorescent protein (EGFP)-expressing USA300 MRSA. Mice were killed 8 h post infection to assess bacterial dissemination; mice in the tamoxifen-treated group exhibited significantly lower bacterial counts in peritoneal lavage fluid as well as in the liver, kidney, spleen and blood ( Fig. 5b ), with bacterial counts below the limit of detection in the tissues of several tamoxifen-treated animals. Analysis of peritoneal lavage fluid using fluorescence microscopy revealed very few intact bacteria in samples from tamoxifen-treated mice, in stark contrast to samples collected from vehicle-treated animals, whose neutrophils contained large numbers of intact bacteria ( Fig. 5c,d ). Of note, neutrophils from these control animals often appeared damaged, consistent with previous findings that S. aureus can promote neutrophil necrosis following phagocytosis [28] . 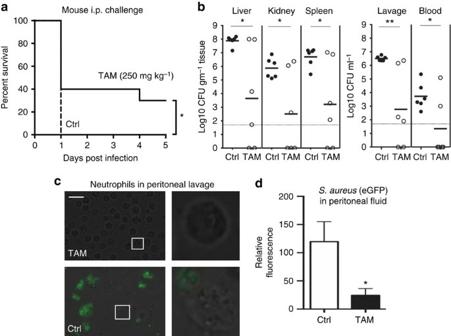Figure 5: Tamoxifen reduces mortality and enhances clearance of USA300 MRSA in anin vivomodel of acute infection. (a) At 1 h following intraperitoneal (i.p.) treatment with tamoxifen (TAM; 250 mg kg−1) or vehicle control (VEH; corn oil), CD-1 background mice were infected i.p. with a lethal dose of USA300 MRSA (5 × 108CFU ml−1, 200 μl). Mice were subsequently treated with tamoxifen or vehicle control at 1 and 8 h post infection and monitored for 5 days. Tamoxifen significantly protected against mortality. (b) To assess bacterial dissemination, CD-1 background mice received i.p. injections of tamoxifen (250 mg kg−1) or vehicle control 2 h before and 6 h following i.p. injection of enhanced green fluorescent protein (EGFP)-expressing USA300 MRSA (5 × 108CFU ml−1, 200 μl). Bacterial counts were determined in the peritoneal lavage fluid and blood, kidney, liver and spleen tissue samples. (c) Light microscopy revealed that neutrophils in the vehicle control samples often appeared damaged and contained multiple intact bacteria (scale bar, 25 μm). (d) Quantitative analysis of fixed peritoneal lavage samples confirmed the presence of elevated EGFP-USA300 MRSA levels in vehicle- versus tamoxifen-treated animals. Results were analysed by the log-rank test (survival curve comparison) or one-way analysis of variance andpost hocNewman Keuls test. *P<0.05, **P<0.01 versus control values. Figure 5: Tamoxifen reduces mortality and enhances clearance of USA300 MRSA in an in vivo model of acute infection. ( a ) At 1 h following intraperitoneal (i.p.) treatment with tamoxifen (TAM; 250 mg kg −1 ) or vehicle control (VEH; corn oil), CD-1 background mice were infected i.p. with a lethal dose of USA300 MRSA (5 × 10 8 CFU ml −1 , 200 μl). Mice were subsequently treated with tamoxifen or vehicle control at 1 and 8 h post infection and monitored for 5 days. Tamoxifen significantly protected against mortality. ( b ) To assess bacterial dissemination, CD-1 background mice received i.p. injections of tamoxifen (250 mg kg −1 ) or vehicle control 2 h before and 6 h following i.p. injection of enhanced green fluorescent protein (EGFP)-expressing USA300 MRSA (5 × 10 8 CFU ml −1 , 200 μl). Bacterial counts were determined in the peritoneal lavage fluid and blood, kidney, liver and spleen tissue samples. ( c ) Light microscopy revealed that neutrophils in the vehicle control samples often appeared damaged and contained multiple intact bacteria (scale bar, 25 μm). ( d ) Quantitative analysis of fixed peritoneal lavage samples confirmed the presence of elevated EGFP-USA300 MRSA levels in vehicle- versus tamoxifen-treated animals. Results were analysed by the log-rank test (survival curve comparison) or one-way analysis of variance and post hoc Newman Keuls test. * P <0.05, ** P <0.01 versus control values. Full size image In sum, we have shown that tamoxifen enhances neutrophil bactericidal activity, with increased NET production a likely contributory mechanism. Our evidence suggests that this enhancement occurs in significant part through the modulation of intracellular ceramide levels. Ceramide, an important bioactive sphingolipid and cellular stress signal, has previously been linked to neutrophil apoptosis [29] , [30] , and tamoxifen-induced ceramide accumulation mediates certain oestrogen receptor-independent effects of the drug against cancer tissues [5] . Here, we show that both tamoxifen and synthetic ceramide are potent inducers of NETosis, a novel cell death pathway with an important role in innate immunity [31] . Interestingly, ceramide can activate both apoptotic and autophagocytic pathways [32] , the latter of which have recently been implicated in NET production [33] . Shifting the balance between apoptotic and autophagocytic pathways may influence relative levels of NET production; indeed, we found that rapamycin, a potent inducer of autophagy, enhanced ceramide-induced NET production while having little effect on its own ( Supplementary Fig. 13 ). Further investigation of compounds that modulate the ceramide biosynthesis pathway may reveal more potent enhancers of neutrophil antimicrobial activity. Along these lines, it is interesting to note that the active metabolite of tamoxifen, 4-hydroxytamoxifen, is even more potent at enhancing NET release and bactericidal activity than tamoxifen. Exploring the mechanism underlying tamoxifen/4-hydroxytamoxifen-induced NET formation may facilitate discovery of derivative compounds specifically optimized to promote targeted enhancement of innate immune responses. The outcomes of enhanced NET production are likely to be pathogen specific. Several bacterial species are capable of evading NET capture through various mechanisms (for example, via the expression of extracellular nucleases capable of cleaving DNA-based structures [34] , [35] ). In the context of S. aureus , a focus of this study, tamoxifen may exhibit particularly marked effects due to the pathogen’s ability not only to evade killing via opsonophagocytosis [36] , [37] and oxidative burst [38] , but also to invade neutrophils and trigger a unique necrolytic pathway. We observed neutrophils in peritoneal lavage samples collected from tamoxifen-treated mice exhibited a significantly reduced bacterial load in comparison with untreated controls. In addition to their role in innate immunity, excessive or aberrant production of NETs has been implicated in inflammatory diseases such as vasculitis and bronchial asthma [39] , [40] . The cumulative effect of tamoxifen on neutrophil responses hold clinical implications, given the large number of patients receiving this drug and related therapeutic agents. Materials Tamoxifen citrate, ceramide, MPP dihydrochloride, G-1, Gö 6983, Gö 6976, PKCζ-PS and DL-PDMP were all obtained from Tocris Bioscience (Bristol, UK). Myriocin was obtained from Cayman Chemical (Ann Arbor, MI). Unless otherwise noted, all other chemicals were obtained from Sigma Aldrich, St Louis, MO. Bacterial strains MRSA strain USA300 (UAMS 1182), E. coli strain K1 and P. aeruginosa strain PA01 were used in this study. EGFP-transformed MRSA strain USA300 (LAC) were used for in vivo studies where indicated. Neutrophil isolation Human venous blood was collected from healthy volunteers, with heparin added as an anticoagulant. Neutrophils were isolated using Polymorphprep (Axis-Shield, Dundee, Scotland) according to the manufacturer’s protocol. Blood was drawn according to a protocol approved by the local ethics committee. Neutrophils were collected from PKCζ knockout animals (C57BL/6 background) and wild-type littermate controls by extracting bone marrow from harvested tibia. Bone marrow was plated on polystyrene dishes and incubated for 37 °C with 5% CO 2 for 1 h; subsequently, neutrophils (still in suspension) were collected, counted and used in experiments. Transwell chemotaxis assay Neutrophils, pre-incubated for 10 min at 24 °C in Hanks' Balanced Salt Solution (HBSS) alone or HBSS with 10 μM tamoxifen, were seeded in 6-mm transwell permeable supports (3 μm pore size; Corning Inc.) that were placed in 24-well plates; lower chambers contained either HBSS alone, or 100 nM fMLP. Following a 45-min incubation at 37 °C, inserts were removed and cells were lysed by addition of Triton X-100 (0.1% final, 10 min, 24 °C). To determine the relative levels of migration to the lower well, the colorimetric elastase substrate N -methoxysuccinyl-Ala-Ala-Pro-Val-p-nitroanilide was added to the lysed cell samples (10 mM final); following a 30-min incubation at 24 °C, absorbance at 405 nm was measured using a SpectraMAX Gemini EM fluorescence reader (Molecular Devices, Sunnyvale, CA). Induction and quantification of NETs To induce extracellular trap production, neutrophils were seeded in 96-well plates at a density of 2 × 10 5 cells per well in HBSS (final volume: 200 μl). Where applicable, cells were incubated with NETosis inhibitors at 37 °C with 5% CO 2 for 60 min (myriocin), 45 min (PKCζ-PS) or 30 min (all other inhibitors) before addition of NET-inducing agents. NET inducers were then added, and cells were incubated for a further 2 h at 37 °C with 5% CO 2 . Where applicable, 25 nM PMA was included as a positive control. Micrococcal nuclease was then added (final concentration: 500 mU ml −1 ) before an additional 10-min incubation at 37 °C. Micrococcal nuclease activity was stopped via the addition of 5 mM EDTA, and plates were spun at 200 g for 8 min. Supernatant samples (100 μl) were collected from each well, and extracellular DNA content was quantified using a Quant-IT PicoGreen dsDNA Assay kit (Life Technologies, Carlsbad, CA) according to the manufacturer’s instructions. NET visualization and fluorescence microscopy To visualize NETs, cells were seeded on 24-well plates at a density of 2 × 10 5 cells per well. Following stimulation of NET production (2 h, 37 °C with 5% CO 2 with indicated drugs), cells were fixed by the addition of paraformaldehyde (4% final) for 10 min at 24 °C. After blocking for 45 min with PBS containing 2% bovine serum albumin (2% PBS–BSA) and 2% goat serum, cells were immunostained via the following incubation steps (each at room temperature): 1 h with rabbit anti-human myeloperoxidase primary antibody (1:300 in 2% PBS–BSA; Dako North America, Inc., Carpinteria, CA; cat # A039829-2), 45 min (protected from light) with Alexa Fluor 488 goat anti-rabbit immunoglobulin G secondary antibody (1:500 in 2% PBS–BSA); Life Technologies, cat # A11070) and 10 min with 1 μM Hoechst-33342-trihydrochloride. Three washes with PBS were performed after each staining step. Images were obtained using a Zeiss AxioObserver D1 microscope equipped with an LD A-Plan × 20/0.35 Ph1 objective. Imaging of intracellular ceramide was performed by permeabilizing cells with 0.25% Triton X-100 following fixation with paraformaldehyde, blocking with 2% PBS–BSA and 2% donkey serum for 1 h, followed by incubation for 1 h with mouse anti-ceramide primary antibody (1:300 in 2% PBS–BSA; Sigma Aldrich; cat # C8104-50TST) and 45 min (protected from light) with Alexa Fluor 488 donkey anti-mouse immunoglobulin G secondary antibody (1:500 in 2% PBS–BSA; Life Technologies; cat # A21202). Representative images shown were collected the Zeiss AxioObserver D1 microscope and objective described above, with exposure and gain settings kept consistent during collection of control and tamoxifen-treated images. A similar protocol in combination with a PKCζ primary antibody (1:200 in 2% PBS–BSA; Abcam, Cambridge, MA, cat # ab59364) was used to visualize intracellular PKCζ distribution using a Leica TCS SPE confocal microscope equipped with a HC PLAN APO × 63/1.40–0.60 numerical aperture oil immersion objective. For live/dead cell analysis, neutrophils were incubated in eight-well LabTek II glass-bottom slides (Nalge Nunc, Penfield, NY) for 2 h with or without tamoxifen, followed by addition of USA300 MRSA (multiplicity of infection (MOI): 5). After 30 min, cells were stained using a LIVE/DEAD BacLight Bacterial Viability kit according to the manufacturer’s instructions. Cells were fixed with 4% paraformaldehyde and imaged using the Leica TCS SPE confocal microscope and objective described above. ROS production assays Neutrophils were incubated in HBSS containing 10 μM 2′,7′-dichlorofluorescein diacetate for 20 min at 37 °C with gentle agitation. Neutrophils were then centrifuged at 400 g for 5 min, washed with HBSS and centrifuged again using the same settings before being counted and resuspended in HBSS at a concentration of 5 × 10 6 cells per ml. Samples of the cell suspension were then added to a 96-well plate (5 × 10 5 cells per well) and mixed at a 1:1 ratio with PMA, ceramide, tamoxifen or 4-hydroxytamoxifen. Fluorescence intensity (485 nm excitation, 530 nm emission) was measured in 15-min intervals using a SpectraMAX Gemini EM fluorescence reader over the course of 2 h (plates were incubated at 37 °C, protected from light and with gentle shaking, between reads). Extraction and quantification of ceramide species Cellular lipids were extracted from neutrophils using the protocol described by Zhang et al . [41] Samples obtained from these extractions were analysed using Orbitrap Fusion Tribrid mass spectrometry technology. Briefly, nano ultra-HPLC was performed on a Thermo Fisher EASY-nLC (Thermo Fisher Scientific Inc., Waltham, MA) with an incorporated cooled autosampler compartment calibrated for a 6 × 8-sample grid. The flow rate was set to 300 nl min −1 , and an 85-min gradient was run. Mobile phase A consisted of 0.1% formic acid in water and mobile phase B consisted of 0.1% formic acid in acetonitrile. The nano-analytical column was prepared by pulling Polymicro fused silica, 30 cm × 75 μm, (Polymicro Technologies, Phoenix, AZ) and packing with 3 μm UChrom C18 bulk-packing material (nanoLCMS Solutions LLC). Analysis was performed on a finely calibrated Thermo Fisher Orbitrap Fusion Tribrid mass spectrometer (Thermo Fisher Scientific Inc.). Positive electrospray ion mode was used in all runs in the targeted selective ion-monitoring scan mode. Relative quantification of the structurally confirmed ceramide species was determined by integration of the peak areas obtained from the extracted ion chromatogram using Xcalibur software. Bacterial growth curves Glass tubes containing Todd Hewitt broth plus vehicle (10% HBSS), tamoxifen (10 μM) or 4-hydroxytamoxifen (10 μM) were inoculated with sufficient amounts of overnight bacterial cultures to achieve an optical density (600 nm) of 0.1. Tubes were incubated in a shaking 37 °C incubator, and absorbance measurements at 600 nm were taken every hour up to 7 h, and once at 24 h, using a Spectronic 20D+ spectrophotometer (Thermo Scientific, Waltham, MA, USA). In vitro bactericidal assays Freshly isolated neutrophils in serum-free RPMI were added to 48-well plates at a density of 4 × 10 5 cells per well. HBSS, tamoxifen or 4-hydroxytamoxifen was added to applicable wells, resulting in a final volume of 200 μl, and cells were incubated for 4 h at 37 °C with 5% CO 2 (identical wells containing no neutrophils were also prepared). Overnight cultures of bacteria were resuspended in RPMI containing 10% 70 °C heat-inactivated fetal bovine serum to achieve a density of 8 × 10 5 CFUs per ml. Fifty microlitre of this bacterial suspension was added to applicable wells of the 48-well plate, resulting in a 2% final concentration of fetal bovine serum and a MOI of 0.1. Plates were then centrifuged at 1,600 r.p.m. for 5 min before a 15-min incubation at 37 °C. A total of 25 μl was then collected from each well and serially diluted in a 96-well plate containing sterile water (225 μl per well). Samples (25 μl) from each well were collected and plated on Todd Hewitt agar (THA) plates, which were incubated at 37 °C overnight. Colonies were counted the next day to calculate bacterial survival. For bactericidal assays using opsonized bacteria, USA300 MRSA were incubated for 30 min in 80% 56 °C heat-inactivated pooled human serum in RPMI before being combined with neutrophils in a 96-well plate (such that the final concentration of serum was 2% and the MOI was 1). Samples were collected, serially diluted in water and plated on THA plates to quantify CFUs. Phagocytosis assay Neutrophils were combined in a 96-well plate (2 × 10 5 cells per well) with pHrodo Red S. aureus Bioparticles (Life Technologies) as specified by the manufacturer. Plates were incubated at 37 °C, and phagocytosis was assessed by measuring fluorescence intensity (560 nm excitation, 585 nm emission) at 15-min intervals using a SpectraMAX Gemini EM fluorescence reader (Molecular Devices). Murine infection studies For in vivo infection studies, 8-week-old female CD-1 mice (Charles River Laboratories, Wilmington, MA, USA) were injected intraperitoneally with tamoxifen (250 mg kg −1 ) or vehicle (corn oil) ( n =6 mice per group). After an hour, mice were infected intraperitoneally with a lethal dose ( ∼ 1 × 10 9 CFU) of MRSA strain USA300 (UAMS 1182). The mice received additional tamoxifen or vehicle treatments 1 and 8 h following infection, and survival was monitored over 7 days. Mice that appeared moribund were humanely killed. To determine CFUs in tissues of tamoxifen-treated and control animals, mice were treated with tamoxifen or vehicle 2 h before and 6 h after i.p. infection with EGFP-expressing USA300 MRSA. Mice were killed 8 h post infection. Peritoneal lavage and blood samples were collected along with the kidneys, livers and spleens of the infected animals. Following homogenization of organs using a MagNA Lyser instrument (Roche Diagnostics Corporation, Indianapolis, IN), samples were serially diluted in PBS and plated on THA plates to determine CFUs per gram of tissue. Two hundred-microlitre samples of the peritoneal lavages were fixed via addition of 4% paraformaldehyde and imaged using the Zeiss AxioObserver system described above. This in vivo infection study was performed in duplicate, and data from one representative experiment are shown. All studies involving animals were reviewed and approved by the University of California San Diego Animal Care and Use Committee. Statistical analysis All of the statistical analyses described in the figure legends were performed using Prism v6.0. Unless otherwise noted, n values indicate the number of replicates performed in at least three independent experiments. How to cite this article: Corriden, R. et al . Tamoxifen augments the innate immune function of neutrophils through modulation of intracellular ceramide. Nat. Commun. 6:8369 doi: 10.1038/ncomms9369 (2015).